Stimulated emission depletion-based raster image correlation spectroscopy reveals biomolecular dynamics in live cells Raster image correlation spectroscopy is a powerful tool to study fast molecular dynamics such as protein diffusion or receptor–ligand interactions inside living cells and tissues. By analysing spatio-temporal correlations of fluorescence intensity fluctuations from raster-scanned microscopy images, molecular motions can be revealed in a spatially resolved manner. Because of the diffraction-limited optical resolution, however, conventional raster image correlation spectroscopy can only distinguish larger regions of interest and requires low fluorophore concentrations in the nanomolar range. Here, to overcome these limitations, we combine raster image correlation spectroscopy with stimulated emission depletion microscopy. With imaging experiments on model membranes and live cells, we show that stimulated emission depletion-raster image correlation spectroscopy offers an enhanced multiplexing capability because of the enhanced spatial resolution as well as access to 10–100 times higher fluorophore concentrations. Live-cell fluorescence microscopy yields unprecedented insight into functionally important biomolecular processes as they occur in space and time. The field has enjoyed rapid progress, thanks to advances in fluorescence marker and labelling techniques, as well as microscopy hardware and analysis tools [1] . In addition to straightforward imaging of slow dynamics, an extensive toolbox of quantitative methods has been established to observe fast molecular motions. Fluorescence recovery after photobleaching [2] , for example, measures molecular mobility by introducing a sudden perturbation to the sample, that is, by applying a localized bleaching pulse. The subsequent relaxation back to equilibrium is observed as a recovery of the fluorescence signal. Other techniques, such as fluorescence correlation spectroscopy (FCS) [3] and raster image correlation spectroscopy (RICS) [4] , rely on the presence of spontaneous fluctuations of the fluorescence, which can arise from the statistically varying population of fluorophores due to their diffusion into and out of the observation volume. These methods require a high detection sensitivity but no perturbation of the system. However, the study of fluctuations is more subtle because their amplitudes are only sufficiently large if the number of observed molecules is small on average. FCS and RICS measurements are usually performed with a confocal microscope. It provides an observation volume of typically ~1 fl, defined by the lateral confinement of light tightly focused by a high-numerical aperture objective and the axial confinement resulting from the presence of a confocal pinhole or two-photon excitation. Even with such a tiny volume, highly dilute fluorophores (in the nanomolar concentration range) are needed. This requirement poses a severe limitation for live-cell studies, in which fluorophore concentration and background signals cannot be well controlled. Here we have applied stimulated emission depletion (STED) microscopy to RICS to overcome these limitations. The use of STED-RICS allows the observation volume to be significantly decreased, so that measurements are feasible with 10–100 times higher fluorophore concentrations than in standard RICS. Unlike FCS, which is a local probe of dynamics, RICS is based on imaging, so that different regions of a heterogeneous sample, for example, cells or tissues, can be probed in parallel. The higher spatial resolution of STED-RICS enables dynamics within smaller regions to be studied. We illustrate the advantages of the new method with measurements on model membranes and live cells. The STED-RICS method In a static FCS experiment, fluorescently labelled molecules diffuse freely through a confocal volume that is held at a fixed position, while the fluorescence intensity is continuously monitored over time ( Fig. 1a , left). From these data, the autocorrelation of the fluorescence intensity, G ( τ ), is computed for different lag times, τ ( Fig. 1b ). The amplitude of G ( τ ) yields the fluorophore concentration; its temporal decay is a measure of the fluorophore mobility in the focal spot. By applying a suitable model, the diffusion coefficient, D , can be computed. Obviously, for homogeneous samples, the point of observation is irrelevant. When studying heterogeneous samples, for example, the cellular interior, however, the observation volume has to be positioned into multiple, precisely defined spots to explore variations in the dynamics. Such static FCS experiments can get cumbersome due to data acquisition at one spot after the other. Moreover, conditions may change during the course of the experiment, and cell movements may generate misplacements, which may even go unnoticed. 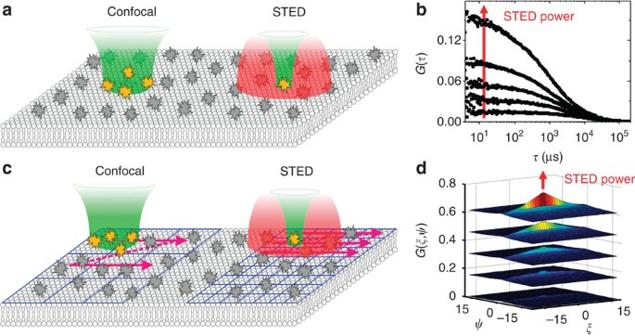Figure 1: Principles of STED-FCS and STED-RICS. (a) In a static confocal FCS measurement (left), the confocal observation volume is placed into a region of interest within the sample, and fluctuations in fluorescence intensity resulting from molecular dynamics are monitored. By using STED-FCS (right), the observation volume can be significantly decreased in a controlled fashion. (b) The amplitude of the intensity autocorrelation function increases because fewer molecules are probed in an observation volume that decreases in size with increasing STED beam power. The dynamics of the fluorophores can be quantified by analysing the temporal decay. (c) In a confocal RICS measurement (left), the observation volume is scanned across the sample in a temporally controlled manner to measure intensities pixel by pixel, so images are acquired that are analysed afterwards. By using STED (right), the observation volume can be significantly decreased in a controlled fashion. Consequently, much finer scan steps can be applied, yielding super-resolution images. (d) Because each pixel and each line are acquired with well-defined mutual time delays, a two-dimensional spatial correlation function calculated for a sub-region yields dynamic information comparable to an FCS experiment; data from all sub-regions can be joined to form a mobility map. As for STED-FCS, increasing the STED power decreases the observation volume and, thereby, increases the correlation amplitudes. The data shown inbanddwere measured on a lipid bilayer. Figure 1: Principles of STED-FCS and STED-RICS. ( a ) In a static confocal FCS measurement (left), the confocal observation volume is placed into a region of interest within the sample, and fluctuations in fluorescence intensity resulting from molecular dynamics are monitored. By using STED-FCS (right), the observation volume can be significantly decreased in a controlled fashion. ( b ) The amplitude of the intensity autocorrelation function increases because fewer molecules are probed in an observation volume that decreases in size with increasing STED beam power. The dynamics of the fluorophores can be quantified by analysing the temporal decay. ( c ) In a confocal RICS measurement (left), the observation volume is scanned across the sample in a temporally controlled manner to measure intensities pixel by pixel, so images are acquired that are analysed afterwards. By using STED (right), the observation volume can be significantly decreased in a controlled fashion. Consequently, much finer scan steps can be applied, yielding super-resolution images. ( d ) Because each pixel and each line are acquired with well-defined mutual time delays, a two-dimensional spatial correlation function calculated for a sub-region yields dynamic information comparable to an FCS experiment; data from all sub-regions can be joined to form a mobility map. As for STED-FCS, increasing the STED power decreases the observation volume and, thereby, increases the correlation amplitudes. The data shown in b and d were measured on a lipid bilayer. Full size image Here, RICS, a method conceptually closely related to FCS, is advantageous. It is based on the acquisition of raster-scanned images, so the sample is continuously imaged throughout the experiment. Therefore, cell movements can be tracked, and regions can be selected for analysis after data acquisition. In addition, fluorescence from immobile objects can be removed. By using RICS, the observation volume is moved across the sample in a temporally controlled fashion ( Fig. 1c , left, scanning indicated by arrows), so that each image contains a time structure determined by the pixel and line dwell times. Subsequently, the pixel intensities are correlated pixel by pixel, with inter-pixel distance, ξ , and line by line, with inter-line distance, ψ , to yield a two-dimensional correlation function, G ( ξ , ψ ) ( Fig. 1d ). With suitably chosen pixel size and dwell times, G ( ξ , ψ ) reveals the mobility of molecules within sub-regions of the image. Two characteristic time scales are utilized for probing fast dynamics, the pixel-to-pixel (microsecond) and the line-to-line (millisecond) delay times. Thus, a mobility map can be computed with a resolution that is a bit lower than the optical resolution. By using this multiplexing approach, protein complexes were studied in cell adhesions in a spatially resolved manner [5] . As an added benefit, as with other scanning fluorescence correlation methods [6] , [7] , such as line scanning FCS [8] or circle scanning FCS [9] , immobile fractions can be identified and eliminated in RICS analysis [10] . The usefulness of FCS and RICS can be greatly enhanced by further reduction of the observation volume, for example, by using laser-induced STED, which forms the basis of STED microscopy [11] , [12] . Based on a confocal setup, the excitation beam is overlaid with a second, red-shifted beam inducing stimulated emission of electronically excited fluorophores ( Fig. 1a , right). Appropriate phase modulation of this depletion beam produces an intensity zero in the centre of the focal spot, flanked by a non-linear increase in depletion intensity ( Supplementary Fig. S1 ). Thus, only fluorophores within the central region escape deexcitation and can spontaneously emit fluorescence photons that are registered by the detector. The STED-induced spatial confinement determines the size of the observation volume, and can be adjusted via the intensity of the STED beam. The higher the STED power, the smaller the observation volume, and the fewer fluorophores within this volume give rise to larger fluctuations and, therefore, greater correlation amplitudes ( Fig. 1b , arrows). Thereby, the usable fluorophore concentration range of STED-FCS is extended by a factor of 10–100, and the improved spatial resolution provides access to dynamics on smaller spatial scales [13] , [14] . As for STED-FCS, the extension of the usable concentration range is a key advantage of STED-RICS. In addition, the spatial resolution of the mobility map is significantly enhanced, enabling a dynamic analysis within regions with lateral dimensions of a few hundred nanometres. Probing lipid dynamics in a model membrane by STED-RICS To evaluate the performance of STED-RICS with our home-built STED microscope ( Supplementary Fig. S1 ), we have employed a lipid bilayer on a solid support as a model system for a biological membrane. It was sparsely labelled with the dye Atto647N conjugated to 1,2-dipalmitoyl- sn -glycero-3-phosphoethanolamine (Atto647N-DPPE) to observe lipid diffusion at 24 °C. A region of 2 × 8 μm 2 (256 × 1024 pixels) was imaged repeatedly (20 frames, 8 μs pixel dwell time, 2.1 ms line repetition time) using 640-nm fluorescence excitation and a 780-nm STED beam at varying powers. In confocal mode (that is, STED beam power zero), the fluorescence intensity fluctuations are dominated by photon shot noise giving rise to a granular structure of the scan image ( Fig. 2a , upper left). Despite the sparse labelling, there are many fluorophores within the confocal spot on average, so the contribution from fluorophore number changes to the intensity fluctuations is small. By using STED, the effective size of the observation volume can be significantly decreased ( Supplementary Fig. S2 ). With fewer markers in the observation volume, large relative number fluctuations due to molecular diffusion into and out of the volume occur, which strongly modulate the fluorescence intensity. Characteristic streaks are observed in the image, which result from an incidental agreement of the motion direction of one or more markers with the scanning direction, temporarily increasing the local marker concentration ( Fig. 2a , lower right). Eight sub-regions (128 × 128 pixels) were extracted from the data sets recorded in confocal mode and with nine different STED powers. Correlation analysis of each data set and fitting with a free diffusion model ( Fig. 3 ) yielded the marker density, 261±5 μm −2 , and the diffusion coefficient, 3.0±0.4 μm 2 s −1 . As shown in Fig. 2b , respectively, the average numbers of molecules and average transit times decrease linearly with the focal area, precisely controllable via the STED intensity ( Supplementary Fig. S3 ). We note that the error bars in Fig. 2c decrease with the focal area because the precision of a STED-RICS experiment improves due to the enhancement of fluctuations. Thus, by proper choice of the STED power, STED-RICS offers the possibility to adjust the optimal observation volume for a given sample. With the smallest observation volume (STED power 200 mW), we obtained a diffusion coefficient of 2.7±0.5 μm 2 s −1 as an average over eight measurements ( Fig. 4 ), which agrees well with values that we determined by static FCS (3.4±0.9 μm 2 s −1 ) and fluorescence recovery after photobleaching (2.9±0.4 μm 2 s −1 ) experiments ( Supplementary Figs S4 and S5 ) and with the value of 3.5±0.3 μm 2 s −1 from the literature for a similar sample [15] . 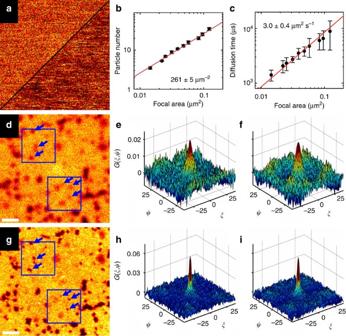Figure 2: Comparison of RICS and STED-RICS applied to a lipid bilayer on a solid support labelled with Atto647N-DPPE. (a) The scan image of the bilayer in confocal mode (upper left) shows only intensity fluctuations due to photon shot noise; number fluctuations of fluorophores do not contribute significantly because of the high lipid marker density used here. By using 200 mW of STED (lower right), the observation volume is significantly reduced (to less than a tenth of its normal lateral size), and horizontal stripes caused by diffusion of individual Atto647N-DPPE lipids are visible. (b) Several image stacks of the same membrane region were recorded at various STED powers and analysed by means of the RICS method. The number of fluorophores was extracted from the amplitudes of the RICS correlation functions by fitting them with a two-dimensional diffusion model (see Methods) and plotted against the (STED power-dependent) focal area, which was determined by calibration measurements (Supplementary Fig. S3). A linear fit yielded an average marker density of 261±5 μm−2. (c) The diffusional correlation time also depends linearly on the focal area, resulting in a diffusion coefficient of 3.0±0.4 μm2s−1for Atto647N-DPPE in the model membrane at 24 °C. Note that the error bars (s.d.) decrease with increasing STED power. (d) Confocal image of a bilayer region containing local defects, some of which are marked by blue arrows. (e,f) RICS correlation functions of the upper and lower (64 × 64 pixels) sub-regions marked by blue squares ind, respectively. (g) STED image from the same region, acquired with a STED power of 60 mW, showing much better resolved local defects. (h,i) STED-RICS correlation functions of the upper and lower sub-regions marked by blue squares ing, respectively. Much better sampling of the STED-RICS data results in better statistics and suppressed artificial long-range correlations in comparison with the confocal RICS data. Scale bars, 1 μm. Figure 2: Comparison of RICS and STED-RICS applied to a lipid bilayer on a solid support labelled with Atto647N-DPPE. ( a ) The scan image of the bilayer in confocal mode (upper left) shows only intensity fluctuations due to photon shot noise; number fluctuations of fluorophores do not contribute significantly because of the high lipid marker density used here. By using 200 mW of STED (lower right), the observation volume is significantly reduced (to less than a tenth of its normal lateral size), and horizontal stripes caused by diffusion of individual Atto647N-DPPE lipids are visible. ( b ) Several image stacks of the same membrane region were recorded at various STED powers and analysed by means of the RICS method. The number of fluorophores was extracted from the amplitudes of the RICS correlation functions by fitting them with a two-dimensional diffusion model (see Methods) and plotted against the (STED power-dependent) focal area, which was determined by calibration measurements ( Supplementary Fig. S3 ). A linear fit yielded an average marker density of 261±5 μm −2 . ( c ) The diffusional correlation time also depends linearly on the focal area, resulting in a diffusion coefficient of 3.0±0.4 μm 2 s −1 for Atto647N-DPPE in the model membrane at 24 °C. Note that the error bars (s.d.) decrease with increasing STED power. ( d ) Confocal image of a bilayer region containing local defects, some of which are marked by blue arrows. ( e , f ) RICS correlation functions of the upper and lower (64 × 64 pixels) sub-regions marked by blue squares in d , respectively. ( g ) STED image from the same region, acquired with a STED power of 60 mW, showing much better resolved local defects. ( h , i ) STED-RICS correlation functions of the upper and lower sub-regions marked by blue squares in g , respectively. Much better sampling of the STED-RICS data results in better statistics and suppressed artificial long-range correlations in comparison with the confocal RICS data. Scale bars, 1 μm. 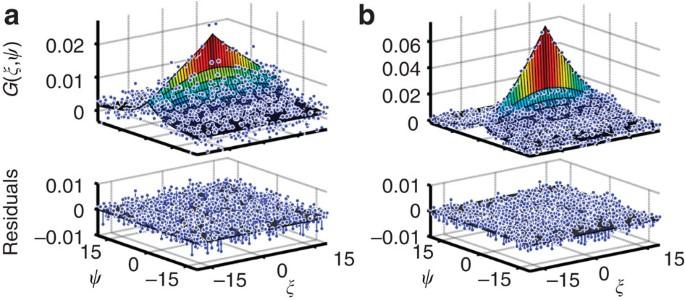Figure 3: Two-dimensional STED-RICS correlation functions on Atto647N-DPPE diffusing in a lipid bilayer. Regions of 256 × 1024 pixels or 256 × 2048 pixels were scanned 10–30 times. From each data set, we extracted sub-micron sized regions of interest for calculation of the image correlation (blue points), followed by fitting (coloured surfaces) with a two-dimensional diffusion model (see Methods). The data were measured with a STED beam power of (a) 16 mW and (b) 100 mW, using a pixel size of 8 nm and a pixel dwell time of 8 μs at 24 °C. Full size image Figure 3: Two-dimensional STED-RICS correlation functions on Atto647N-DPPE diffusing in a lipid bilayer. Regions of 256 × 1024 pixels or 256 × 2048 pixels were scanned 10–30 times. From each data set, we extracted sub-micron sized regions of interest for calculation of the image correlation (blue points), followed by fitting (coloured surfaces) with a two-dimensional diffusion model (see Methods). The data were measured with a STED beam power of ( a ) 16 mW and ( b ) 100 mW, using a pixel size of 8 nm and a pixel dwell time of 8 μs at 24 °C. 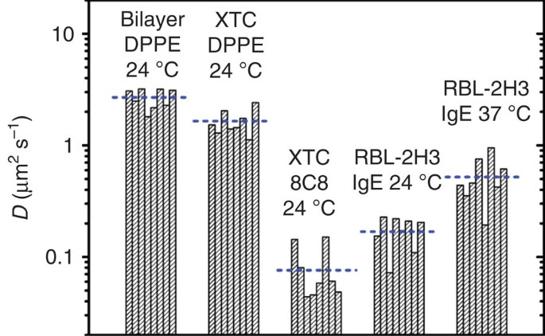Figure 4: Diffusion coefficients obtained by STED-RICS. Compilation of the diffusion coefficients measured in multiple STED-RICS experiments with different samples. Individual measurements are represented by hatched columns; the averages are marked by dashed blue lines. Full size image Figure 4: Diffusion coefficients obtained by STED-RICS. Compilation of the diffusion coefficients measured in multiple STED-RICS experiments with different samples. Individual measurements are represented by hatched columns; the averages are marked by dashed blue lines. Full size image STED-RICS measurements directly benefit from the increase in spatial resolution. The mobility map resolution depends on the image resolution and, therefore, the multiplexing capability is greatly enhanced due to higher spatial sampling achieved by STED-RICS. Like STED-FCS, STED-RICS can reveal particle dynamics on smaller spatial scales than those accessible with diffraction-limited correlation spectroscopy. To illustrate these advantages, we prepared a lipid bilayer with local defects, in which there are no fluorescent markers present. Comparison of the two images taken in confocal and STED modes, Fig. 2d , respectively, reveals that the defects, which are clearly visible as tiny dark spots in STED mode, only appear as blurry, dimmer patches in confocal mode because of the insufficient spatial resolution. RICS analysis yields the average particle mobility within chosen sub-regions, such as the two sub-regions of 64 × 64 pixels (2 × 2 μm 2 ) marked in Fig. 2d by blue boxes. In the correlation functions, G ( ξ , ψ ), calculated from the confocal images ( Fig. 2e ), these local variations appear as artificial long-range correlations, causing problems for the quantitative analysis. In STED mode, the statistics of G ( ξ , ψ ) is significantly improved because of the much better sampling due to the higher resolution ( Fig. 2h ). Thus, artificial long-range correlations are suppressed in the correlation function, enabling a reliable data analysis. Live-cell dynamics studied by STED-RICS We further compared STED-RICS and conventional RICS by performing experiments on three different live-cell samples. An important application of RICS is the study of receptor–ligand interactions at the cell membrane. To this end, we added IgE molecules labelled with Atto647N to live RBL-2H3 mast cells, to which they bind via the high-affinity IgE receptor (FcεRI) in the plasma membrane. In the overview image in Fig. 5a , the region marked by the white rectangle is also displayed as a close-up STED image and a regular confocal image. It shows that the bound complex is not homogeneously dispersed over the cell membrane, but rather concentrated in patches of high local concentration. Image correlation was straightforward using STED-RICS ( Fig. 5b ), whereas confocal RICS analysis was not possible under our experimental conditions ( Fig. 5c ). To further strengthen the evidence, we performed STED-RICS experiments at two different temperatures, 24 and 37 °C, yielding average diffusion coefficients of 0.17±0.06 and 0.5±0.2 μm 2 s −1 , respectively. As expected, the dynamics accelerates with temperature. These data are also included in Fig. 4 . 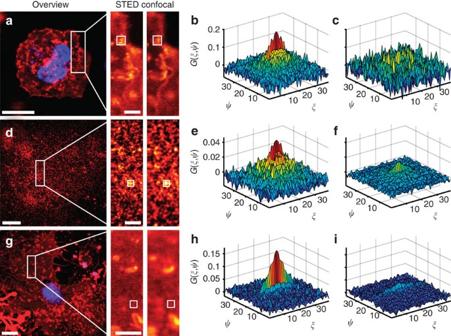Figure 5: Three examples of live-cell applications of STED-RICS. Data for RICS analysis were acquired by using pixel sizes, dwell times and STED intensities optimally chosen for the different dynamics of the samples. (a) Overview fluorescence image of an RBL-2H3 mast cell labelled with Hoechst 33258 (blue nuclear stain, excited via 780-nm two-photon absorption) and Atto647N-labelled IgE (red channel) binding to FcεRI (membrane, red). A close-up is provided in STED and confocal modes, as well as (b) STED-RICS and (c) RICS correlation functions from the sub-region (62 × 62 pixels) marked by a white square in the close-ups. For FcεRI diffusing in the membrane of RBL-2H3 mast cells (D=0.5±0.2 μm2s−1, 37 °C), a pixel size of 16 nm, a dwell time of 10 μs and a STED intensity of 200 mW were found optimal. (d) Overview fluorescence image of an XTC cell immunostained with monoclonal anti-β1-integrin IgG 8C8 labelled with Atto647N (red). Again, close-ups of the sub-region marked by a white rectangle are shown in STED and confocal modes, and (e) STED-RICS and (f) RICS correlation functions from the sub-region (38 × 38 pixels) marked by a white square in the close-ups. To capture the much slower dynamics of β1-integrin on XTC cells (D=0.08±0.04 μm2s−1, 24 °C), we used a pixel size of 16 nm, dwell time of 20 μs and STED intensity of 100 mW. (g) Overview fluorescence image of XTC cells labelled with Hoechst 33258 (blue nuclear stain, excited via 780-nm two-photon absorption) and Atto647N-DPPE-BSA (membrane, red). Close-up images of the sub-region marked by a white rectangle are again shown in STED and confocal modes. (h) STED-RICS and (i) RICS correlation functions from the sub-region (50 × 50 pixels) marked in the close-ups by a white square. A pixel size of 10 nm, dwell time of 10 μs and STED intensity of 200 mW were used for measuring the fast diffusion of Atto647N-DPPE-BSA in the XTC cell membrane (D=1.6±0.4 μm2s−1, 24 °C). Scale bars, 10 μm (overview) and 2 μm (close-ups). Figure 5: Three examples of live-cell applications of STED-RICS. Data for RICS analysis were acquired by using pixel sizes, dwell times and STED intensities optimally chosen for the different dynamics of the samples. ( a ) Overview fluorescence image of an RBL-2H3 mast cell labelled with Hoechst 33258 (blue nuclear stain, excited via 780-nm two-photon absorption) and Atto647N-labelled IgE (red channel) binding to FcεRI (membrane, red). A close-up is provided in STED and confocal modes, as well as ( b ) STED-RICS and ( c ) RICS correlation functions from the sub-region (62 × 62 pixels) marked by a white square in the close-ups. For FcεRI diffusing in the membrane of RBL-2H3 mast cells ( D =0.5±0.2 μm 2 s −1 , 37 °C), a pixel size of 16 nm, a dwell time of 10 μs and a STED intensity of 200 mW were found optimal. ( d ) Overview fluorescence image of an XTC cell immunostained with monoclonal anti-β1-integrin IgG 8C8 labelled with Atto647N (red). Again, close-ups of the sub-region marked by a white rectangle are shown in STED and confocal modes, and ( e ) STED-RICS and ( f ) RICS correlation functions from the sub-region (38 × 38 pixels) marked by a white square in the close-ups. To capture the much slower dynamics of β1-integrin on XTC cells ( D =0.08±0.04 μm 2 s −1 , 24 °C), we used a pixel size of 16 nm, dwell time of 20 μs and STED intensity of 100 mW. ( g ) Overview fluorescence image of XTC cells labelled with Hoechst 33258 (blue nuclear stain, excited via 780-nm two-photon absorption) and Atto647N-DPPE-BSA (membrane, red). Close-up images of the sub-region marked by a white rectangle are again shown in STED and confocal modes. ( h ) STED-RICS and ( i ) RICS correlation functions from the sub-region (50 × 50 pixels) marked in the close-ups by a white square. A pixel size of 10 nm, dwell time of 10 μs and STED intensity of 200 mW were used for measuring the fast diffusion of Atto647N-DPPE-BSA in the XTC cell membrane ( D =1.6±0.4 μm 2 s −1 , 24 °C). Scale bars, 10 μm (overview) and 2 μm (close-ups). Full size image We also applied STED-RICS to the study of focal adhesion dynamics. In previous work, we observed assembly and disassembly of individual focal adhesions by using super-resolution PALM imaging combined with pulse-chase experiments, based on the photoactivatable fluorescent protein mIrisFP fused to paxillin [16] . Here we have investigated focal adhesions of Xenopus laevis tissue culture (XTC) cells using β1-integrin, immunostained with the monoclonal antibody 8C8 labelled with Atto647N ( Fig. 5d ). After the cells adhered to the surface, RICS data were recorded in areas of 4 × 16 μm 2 (256 × 1024 pixels, 16 nm pixel size, 20 μs pixel dwell time). We performed a STED-RICS analysis of a sub-region of 640 × 640 nm 2 marked by white boxes in the close-ups in Fig. 5d covering an individual focal contact of sub-micron size. We found a very slow dynamics for β1-integrin, with a diffusion coefficient of 0.08±0.04 μm 2 s −1 at 24 °C ( Fig. 4 ), which is also apparent from the considerable width of G ( ξ , ψ ) along the ψ axis, indicating a strong line-to-line correlation ( Fig. 5e ). In contrast, G ( ξ , ψ ) from the confocal RICS data is not suitable for quantitative analysis ( Fig. 5f ). Furthermore, we labelled the plasma membrane of XTC cells using Atto647N-DPPE in a complex with BSA. We performed the correlation analysis for a sub-region of 640 × 640 nm 2 marked by white boxes in the close-ups in Fig. 5g . The correlation functions G ( ξ , ψ ) are shown in Fig. 5h for STED-RICS and standard RICS, respectively. The analysis of the STED-RICS measurements yields a diffusion coefficient of 1.6±0.4 μm 2 s −1 at 24 °C (also included in Fig. 4 ), whereas confocal RICS analysis fails because the high marker concentration and the small size of the sub-region result in a poor signal-to-noise ratio. In fact, we observed that lipid diffusion in the plasma membrane of live XTC cells could be analysed by using STED-RICS in areas as small as 30 × 30 pixels, that is, 300 × 300 nm 2 for a pixel size of 10 nm. RICS analysis of raster-scanned images provides dynamic information on two characteristic time scales, governed by the pixel-to-pixel and line-to-line time intervals. The pixel dwell time can be chosen at will, but the line dwell time, that is, the time interval between successive lines, scales with the number of pixels in a line. The line-to-line correlation can only contribute to the result if the dynamic process under study is not so fast that the correlation has completely decayed from one line to the next. A suitable line dwell time can, however, be attained by proper choice of the number of pixels in a scan line. Note that the maximum number of lines in a single frame is not limited, assuming that the observed motions are time independent. To achieve a short line repetition time, we image narrow strips instead of square-shaped regions. Data acquisition can be extended in the horizontal direction by dividing a large region of interest into several image strips that are sequentially acquired. As an example of this strategy, we have analysed lipid diffusion in the plasma membrane of live XTC cells within a total area of 18 × 20 μm 2 , split into seven regions of 256 × 2048 pixels ( Fig. 6 ). 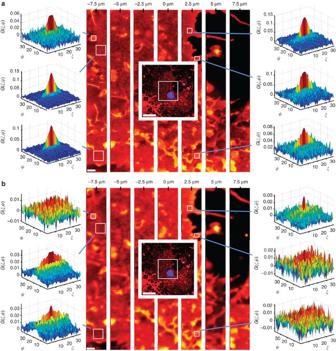Figure 6: Mapping a large region of interest by scanning of narrow strips for STED-RICS analysis. Diffusion of Atto647N-DPPE in the membrane of an XTC cell is mapped by recording seven regions of 256 × 2048 pixels each (10 nm pixel size), resulting in a total observation area of 18 × 20 μm2in (a) STED and (b) confocal modes. An overview of the entire cell is shown in the centres of the middle panels as insets. Scale bars, 20 μm (insets) and 1 μm (strips). RICS correlation functions are shown on the left and right of the images for sub-regions indicated by white rectangles in the middle panels. Figure 6: Mapping a large region of interest by scanning of narrow strips for STED-RICS analysis. Diffusion of Atto647N-DPPE in the membrane of an XTC cell is mapped by recording seven regions of 256 × 2048 pixels each (10 nm pixel size), resulting in a total observation area of 18 × 20 μm 2 in ( a ) STED and ( b ) confocal modes. An overview of the entire cell is shown in the centres of the middle panels as insets. Scale bars, 20 μm (insets) and 1 μm (strips). RICS correlation functions are shown on the left and right of the images for sub-regions indicated by white rectangles in the middle panels. Full size image Optical fluorescence microscopy is a key method to observe biomolecular interactions and dynamics within cells, tissues and entire organisms as they occur in space and time. However, mere imaging often provides only limited insights, and a variety of quantitative fluorescence techniques have been developed to reveal additional information. Among these, fluorescence fluctuation spectroscopy methods have been shown to be particularly powerful [17] . Since the introduction of FCS in 1972 (ref.3) [3] , a wide range of variants have been introduced offering advantages in particular experiments. The recent combination of STED microscopy with FCS was an important advancement because STED allows the observation volume to be decreased by 1–2 orders of magnitude [13] , [14] . Consequently, STED-FCS can accommodate a higher fluorophore concentration than FCS, which is limited to ~1 nM. This is especially helpful for in-vivo experiments, where fluorophore concentration frequently cannot be well controlled. Moreover, the spatial super-resolution of STED microscopy allows smaller regions to be explored. Similarly, the combination of STED with RICS introduced here also benefits from the higher spatial resolution. Both RICS and FCS have their specific strengths, and the choice of method depends on the particular application. FCS has a high temporal resolution, which is only limited by the detector response to typically <1 ns. FCS allows complex dynamics to be followed over a wide time window covering many orders of magnitude. Moreover, single-spot FCS offers the smallest possible observation volume. For RICS, the time resolution depends on the minimum pixel dwell time, which is usually a few microseconds for a conventional confocal beam scanning microscope. Moreover, the time window is not continuous but governed by the pixel and line dwell times, and continuous coverage of a wide time range requires image acquisition with different scan speeds. Because a spatial sub-region is analysed by RICS, the observation volume is larger than for FCS. RICS is based on raster-scan imaging. Therefore, sample movements, for example, cell crawling, are visible and can be taken into account, artifacts such as immobile fractions can be removed from the data at a later stage, and bleaching of slowly moving particles is less of a problem due to the fast-moving beam. Most importantly, however, we can probe dynamics within multiple regions of interest in the sample that can be chosen after data acquisition. This is the key advantage, which makes RICS most useful for live cell and tissue applications. The enhanced optical resolution provided by STED-RICS is particularly beneficial to probe intracellular dynamics over small spatial scales. We note that raster-scan image data can also be subjected to other statistical methods such as number and brightness analysis [18] that likewise benefit from the increased spatial resolution provided by STED. Further technical advancements of STED-RICS can be envisioned in the near future. For example, the temporal resolution may be significantly increased with fast scanners based on acousto-optics rather than galvanometers. Although technically demanding, dual-colour cross-correlation STED-RICS can be implemented to observe interactions between two differently labelled molecules, as is frequently practiced with standard FCS and RICS [5] , [19] . However, already in its basic mode, STED-RICS appears as an elegant and powerful tool for uncovering fast dynamics in live cells and tissues. STED-RICS imaging A schematic of our STED microscope is shown as Supplementary Fig. S1 . Fluorescence is excited by a 640-nm pulsed diode laser (LDH-P-C-640B; PicoQuant, Berlin, Germany), emitting pulses of 100 ps length at a frequency of 80 MHz and an average focal power of 1–6 μW. The excitation light is spectrally cleaned by a 640/14 nm bandpass filter (HC 640/14; Semrock, Rochester, NY, USA) and spatially cleaned by 2 m of single-mode polarization-maintaining fibre (PMC-630; Schäfter+Kirchhoff, Hamburg, Germany). We use an 80-MHz mode-locked Ti:Sa laser (Mai Tai HP; Newport Spectra-Physics, Darmstadt, Germany) tuned to a wavelength of 780 nm for STED using the Atto647N dye. Average STED powers of 50–200 mW efficiently reduce the extension of the observation area to sub-diffractional values (Supplementary Fig. S3). The 100-fs pulse of the Ti:Sa laser is stretched to 200 ps by 60 cm of SF6 glass (AR680-800 SF6; Laser Components, Olching, Germany) followed by 100 m of polarization-maintaining single-mode fibre (PMJ-A3HPC; OZ Optics, Ottawa, Ontario, Canada) [20] . The long STED pulse ensures a complete coverage of the duration of the excitation pulse to efficiently suppress pre-STED fluorescence emission, and minimizes two-photon excitation by the depletion beam. The Ti:Sa pulses are monitored by an internal photodiode, the output of which is used to synchronize the diode laser. To ensure simultaneous arrival of the excitation and depletion pulses, the timing is adjusted by minimizing the fluorescence signal from an Atto647N solution as described [21] . The phase retardation that creates a doughnut-shaped depletion spot is generated by a helical phase plate (VPP-1a; RPC Photonics, Rochester, NY, USA). Excitation and depletion beams are spatially overlaid on a 730-nm shortpass dichroic mirror (z730sprdc; Chroma, Bellow Falls, VT, USA) by measuring the reflection of 80 nm gold beads (GC80; BB International, Dundee, UK) [22] . A quarter-wave plate (RAC 4.4.15; B. Halle, Berlin, Germany) induces circular polarization in the excitation and depletion beams so as to avoid photoselection of the fluorophores and to ensure a high-quality central zero in the doughnut-shaped depletion intensity pattern [21] , [23] . Light is focused into the sample by means of an oil immersion objective (HCX PL APO CS × 100/1.46; Leica, Wetzlar, Germany). Fluorescence light is separated by a quad-band dichroic mirror (zt405/488/561/640rpc; Chroma) and focused into a multimode fibre (M31L02; Thorlabs, Munich, Germany) serving as a confocal pinhole, with the core diameter corresponding to one Airy unit. Subsequently, the fluorescence is filtered by a 700-nm shortpass filter (ET700SP; Chroma) followed by a 676/37 nm bandpass filter (HC 676/37, Semrock) to block scattered excitation and STED photons. Photons are counted by an avalanche photodiode (tau-SPAD-50; PicoQuant) and registered by a data acquisition card (PCI-6259; National Instruments, Munich, Germany). This card also generates the signals controling the laser scanner (Yanus V; Till Photonics, Gräfelfing, Germany). For optimal sampling, the pixel size in a RICS measurement should be 4–5 times smaller than the width of the point spread function [24] , so the optimal pixel size is 8–20 nm for STED-RICS at spatial resolutions of 40–80 nm ( Supplementary Fig. S6 ). The optimal pixel dwell time depends on the average transit time of the molecules through the observation volume, which is governed by the mobility of the molecules and the size of the observation volume. Therefore, STED-RICS requires faster scanning than confocal image acquisition because of the smaller observation volume. We use the software Imspector (Max-Planck-Innovation, Munich, Germany) for image acquisition. A custom-made temperature-controlled sample stage enables experiments at different temperatures. STED-RICS data analysis Correlation analysis of the images is performed using homemade software written in Matlab (MathWorks, Natick, Massachusetts, USA), which is made available as Supplementary Software ( Supplementary Fig. S7 ). After computing the correlation function, G ( ξ , ψ ), we fit the data with the equation: Here, N is the average number of particles within the observation volume and γ =0.35 is a correction factor assuming a three-dimensional Gaussian intensity profile [4] . The term G D ( ξ , ψ ) accounts for free, two-dimensional diffusion, Here, ξ and ψ represent the pixel-to-pixel and line-to-line separations over which the correlations are computed, and τ p and τ 1 are the respective pixel and line dwell times. From the average transit time, τ D , due to particle diffusion, we obtain the diffusion coefficient, D , by using 4 Dτ D = , with ω 0 denoting the width of the observation volume. The scanning term, G S ( ξ , ψ ), accounts for movement of the focal volume during image acquisition [4] , with δ p denoting the pixel size. As suggested previously [13] , we also include a kinetic term, G K ( ξ , ψ ), representing transitions of the dye to a dark state with a lifetime of 30–150 μs for the lipid-dye system [13] . K denotes the amplitude of the kinetic term with dark-state lifetime, τ K . Addition of a triplet term was not needed, presumably because of the minimum pixel dwell time of 8 μs in the STED-RICS measurements, which is above the estimated triplet lifetime of ~3 μs. Lipid bilayer preparation Planar lipid bilayers were prepared by dissolving 1,2-dioleoyl- sn -glycero-3-phosphocholine (Avanti Polar Lipids, Alabaster, AL) and cholesterol (Sigma, Steinheim, Germany) in chloroform at a ratio of 4:1. Atto647N-DPPE (Atto-Tec, Siegen, Germany) was added in the amount of 0.01 mol% to the stock solution (5 mg ml −1 ). Ten microlitres of the lipid solution was evaporated for 1 h under vacuum and afterwards rehydrated with 10 mM HEPES buffer (pH 7.4) containing 150 mM NaCl. The vortexed suspension was sonicated at 60 °C for 1 h, and 100 μl solution was placed in a chamber slide to form the bilayer. Dye conjugation procedures We prepared the Atto647N-DPPE-BSA complex as described [13] . Briefly, a 100 nM Atto647N-DPPE (Atto-Tec) stock solution (CHCl 3 ) was dried under vacuum followed by resuspension in ethanol (20 μl). For complex formation, 1 ml of defatted 100 μM BSA solution in HDMEM (DMEM supplemented with 25 mM HEPES buffer) was added and vortexed vigorously. We added 9 ml HDMEM to yield a final concentration of 10 μM BSA. Both antibodies used in this study, monoclonal anti-β1-integrin IgG 8C8 (Hybridoma Bank, Iowa City, IA, USA) and monoclonal anti-DNP IgE (Sigma) were incubated with Atto647N-NHS (Atto-Tec) for 2 h at 24 °C according to the labelling instructions provided by the manufacturer. The solutions were subsequently purified by gel filtration using Sephadex G-25 columns (Sigma). Cell labelling For studying membrane dynamics, XTC cells attached to chamber slides were incubated for 30 min at 24 °C with the blue nuclear stain Hoechst 33258 (Sigma), followed by incubation on ice with Atto647N-DPPE-BSA for 30 min as described [13] . For studying focal adhesions, XTC cells cultured in frog complete medium for amphibian cells consisting of DMEM supplemented with 30% H 2 O and 10% fetal bovine serum (24 °C and 7% CO 2 ) were detached using 10% chicken serum and 2 mM EDTA. For labelling of β1-integrin, ~10 4 cells were incubated with 8C8-Atto647N (15 μM) for 40 min at 4 °C under constant agitation. Afterwards, the cell suspension was transferred to chamber slides coated with fibronectin. For studying dynamics of the FcεRI complex, RBL-2H3 mast cells cultured in DMEM supplemented with 15% fetal bovine serum at 37 °C, 5% CO 2 and 95% humidity were incubated with IgE-Atto647N (15 μM) for 90 min followed by Hoechst 33258 staining (1 μg ml −1 ) for 30 min. The cells were then collected, washed twice with calcium-free PBS (137 mM NaCl, 2.7 mM KCl, 6.4 mM Na 2 HPO 4 and 1.5 mM KH 2 PO 4 ) and resuspended in Tyrode’s buffer (137 mM NaCl, 2.7 mM KCl, 1 mM MgCl 2 , 1.8 mM CaCl 2 , 0.2 mM Na 2 HPO 4 , 12 mM NaHCO 3 and 5.5 mM D -glucose) with 0.1% BSA. The cell suspension was transferred into chamber slides for further analysis. How to cite this article: Hedde, P. N. et al. Stimulated emission depletion-based raster image correlation spectroscopy reveals biomolecular dynamics in live cells. Nat. Commun. 4:2093 doi: 10.1038/ncomms3093 (2013).